Nedd4-induced monoubiquitination of IRS-2 enhances IGF signalling and mitogenic activity Insulin-like growth factors (IGFs) induce proliferation of various cell types and play important roles in somatic growth and cancer development. Phosphorylation of insulin receptor substrate (IRS)-1/2 by IGF-I receptor tyrosine kinase is essential for IGF action. Here we identify Nedd4 as an IRS-2 ubiquitin ligase. Nedd4 monoubiquitinates IRS-2, which promotes its association with Epsin1, a ubiquitin-binding protein. Nedd4 recruits IRS-2 to the membrane, probably through promoting Epsin1 binding, and enhances IGF-I receptor-induced IRS-2 tyrosine phosphorylation. In thyroid FRTL-5 cells, activation of the cyclic AMP pathway increases the association of Nedd4 with IRS-2, thereby enhancing IRS-2-mediated signalling and cell proliferation induced by IGF-I. The Nedd4 and IRS-2 association is also required for maximal activation of IGF-I signalling and cell proliferation in prostate cancer PC-3 cells. Nedd4 overexpression accelerates zebrafish embryonic growth through IRS-2 in vivo . We conclude that Nedd4-induced monoubiquitination of IRS-2 enhances IGF signalling and mitogenic activity. Insulin-like growth factor (IGF)-I and IGF-II induce cell proliferation, differentiation, survival and migration in many cell types [1] . In vivo , IGFs play important roles in prenatal and postnatal development [2] . Reduced IGF activities cause growth retardation, whereas elevated IGF activities cause overgrowth and cancer development [3] . The growth-promoting activities of IGFs or their homologues are evolutionarily conserved in metazoans [4] . IGFs bind to the IGF-I receptor (IGF-IR) in the plasma membrane and induce the activation of its intrinsic tyrosine kinase and auto-phosphorylation. The activated IGF-IR phosphorylates intracellular substrates including insulin receptor substrate (IRS)-1 and IRS-2. Phosphotyrosyl IRSs are in turn recognized by SH2 domain-containing proteins such as the p85 regulatory subunit of phosphatidylinositol 3-kinase (PI3K). These events trigger activation of downstream signalling pathways, leading to various biological actions [5] . IGF activities are often modulated by other hormonal factors [6] , [7] . IRSs serve as ‘signal nodes’ on which IGF signals and other signals converge. Indeed, IGF-induced IRS tyrosine phosphorylation is potentiated by other hormonal stimuli, leading to amplification of IGF activities [8] , [9] , [10] . In addition, oncogenic pathways frequently cause excess IRS-mediated signalling, which contribute to tumour growth and metastasis [11] . We have shown that IRSs form high-molecular-mass complexes (IRSomes) and different complexes are formed depending on IRS isoform, cell types or hormone stimulation [12] . Subsequent study showed that IRS-associated proteins potentially modulate the availability of IRSs to receptor tyrosine kinases [12] , prompting us to identify IRS-associated proteins and to understand their functions. In this study, we identified HECT-type ubiquitin ligase Nedd4 as a novel IRS-2-associated protein. Nedd4 is expressed in a variety of tissues and regulates the trafficking and/or degradation of its substrate proteins [13] , [14] . IGF-IR is reported to be a putative Nedd4 substrate, but the effects of Nedd4 on IGF-IR are controversial [15] , [16] . Nedd4 knockout mice show fetal growth retardation and perinatal lethality [16] , indicating a crucial role for Nedd4 in embryonic growth. Nedd4 is overexpressed in several types of cancers and functions as an oncogenic protein [17] , [18] , [19] , [20] , [21] . We provide multiple lines of evidence, suggesting that Nedd4 conjugates monoubiquitin to IRS-2 and recruits IRS-2 to the plasma membrane, thereby enhancing IRS-2 tyrosine phosphorylation by IGF-IR and IGF-I mitogenic activity. Nedd4 is an IRS-2-associated protein We previously reported that pretreatment of thyroid FRTL-5 cells with thyroid stimulating hormone (TSH) or other cAMP-generating reagents enhances IGF-I-induced IRS-2 tyrosine phosphorylation and increased cell proliferation [10] , [22] , [23] . Our study also suggested that some IRS-2-associated protein(s) might increase the availability of IRS-2 to the IGF-IR tyrosine kinase [12] . Using co-immunoprecipitation followed by matrix-assisted laser desorption/ionization–time-of-flight mass spectrometry (MS) analysis, we identified Nedd4 as an IRS-2-associated protein in FRTL-5 cells treated with dibutyryl cAMP ( Supplementary Fig. 1a,b ). This association was confirmed by co-immunoprecipitation and immunoblotting ( Supplementary Fig. 1c ). Co-immunoprecipitation analysis using HEK293 cells expressing exogenous IRS-2 together with Nedd4 or Nedd4-2, a related protein in the Nedd4 family [13] , revealed that IRS-2 is associated only with Nedd4 ( Supplementary Fig. 1d ). Next, we generated a series of IRS-2 deletion mutants and performed pull-down analyses. The results revealed that IRS-2 amino acids (aa) 1–134 (containing a PH domain) as well as 137–329 (containing a PTB domain) are critical for its binding to Nedd4 ( Fig. 1a ). Similar experiments using Nedd4 deletion mutants demonstrated that Nedd4 1–226 (containing a C2 domain) is important ( Fig. 1b ). Nedd4 1–226 can bind to IRS-2 1–134 as well as 137–329 in vitro ( Supplementary Fig. 2a ). 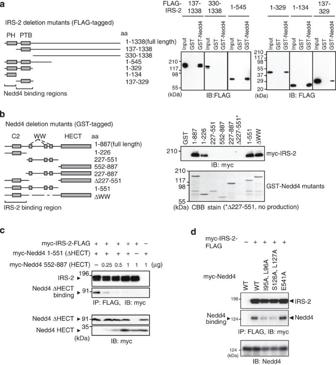Figure 1: Nedd4 is an IRS-2-associated protein. (a,b) Determination of the binding regions. HEK293T cells overexpressing the indicated FLAG-tagged IRS-2 deletion mutants (a) or myc-IRS-2 (b) were serum starved and cell lysates were subjected to pull-down analysis using GST-Nedd4 or its deletion mutants shown inb. The purity of GST-tagged proteins was validated by SDS–PAGE and CBB stain. Input,∼1/100 volume of HEK293T lysates. *GST-Nedd4 Δ227–551 was not successfully expressed. (c,d) Effects of Nedd4 HECT domain (c) and various Nedd4 mutants (d) on the IRS-2–Nedd4 C2 domain interaction. HEK293 cells overexpressing indicated proteins were serum starved and cell lysates were subjected to immunoprecipitation and immunoblotting using the indicated antibodies. Figure 1: Nedd4 is an IRS-2-associated protein. ( a , b ) Determination of the binding regions. HEK293T cells overexpressing the indicated FLAG-tagged IRS-2 deletion mutants ( a ) or myc-IRS-2 ( b ) were serum starved and cell lysates were subjected to pull-down analysis using GST-Nedd4 or its deletion mutants shown in b . The purity of GST-tagged proteins was validated by SDS–PAGE and CBB stain. Input, ∼ 1/100 volume of HEK293T lysates. *GST-Nedd4 Δ227–551 was not successfully expressed. ( c , d ) Effects of Nedd4 HECT domain ( c ) and various Nedd4 mutants ( d ) on the IRS-2–Nedd4 C2 domain interaction. HEK293 cells overexpressing indicated proteins were serum starved and cell lysates were subjected to immunoprecipitation and immunoblotting using the indicated antibodies. Full size image We further investigated the IRS-2-binding site in Nedd4 in greater detail. The Nedd4 C2 domain can bind intramolecularly to the HECT domain [24] . Overexpression of HECT domain in HEK293 cells decreased the association of Nedd4 1–551 with IRS-2 ( Fig. 1c ), indicating that the Nedd4 HECT domain and IRS-2 may competitively bind to the Nedd4 C2 domain. This raised the possibility that the HECT domain and IRS-2 may bind to an overlapping site in the C2 domain. To test this idea, we modelled the Nedd4 intramolecular binding sites based on the reported structure of Smurf2, a Nedd4-type ubiquitin ligase [24] . Based on the modelling results ( Supplementary Fig. 2b ), several mutants were generated. Mutation of Ile 95 and Leu 96 to Ala, or Ser 126 and Leu 127 to Ala inhibited the association of Nedd4 1–502 with Nedd4 503–887 ( Supplementary Fig. 2c ). These data suggest that these residues are part of the intramolecular binding sites. These mutations also inhibited the association of Nedd4 with IRS-2 ( Fig. 1d ), indicating their roles in IRS-2 binding. Nedd4 induces IRS-2 monoubiquitination We investigated whether Nedd4 ubiquitinates IRS-2 using a cell-free ubiquitination assay. The results showed that Nedd4 caused a prominent upward mobility shift of IRS-2, a typical pattern of protein ubiquitination ( Fig. 2a ). Furthermore, overexpression of Nedd4 in HEK293/HEK293T cells increased the ubiquitination signal in IRS-2 immunoprecipitates ( Fig. 2b ). The signal was observed when proteins that bound to IRS-2 (for example, Nedd4) were removed by denaturing the samples before immunoprecipitation ( Fig. 2b ), indicating that the observed signal arose from ubiquitinated IRS-2 itself. The detected signal was 20–30 kDa larger than the intact IRS-2, indicating the conjugation of a small number of ubiquitin molecules. The exact number was unclear, as the IRS-2 mobility may be changed by other posttranslational modifications in addition to ubiquitination. Nedd4-induced IRS-2 ubiquitination was not affected by IGF-I stimulation ( Supplementary Fig. 3a ). Nedd4 overexpression also induced IGF-IR ubiquitination as previously reported [15] , but it did not induce IRS-1 ubiquitination ( Supplementary Fig. 3a ). 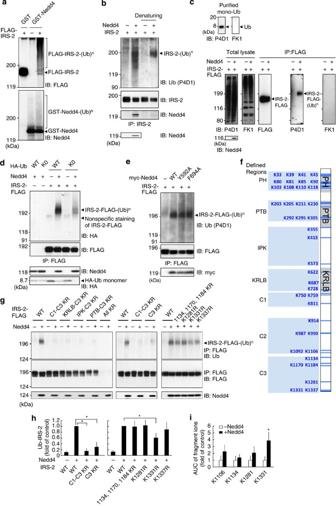Figure 2: Nedd4 induces IRS-2 monoubiquitination. (a) Cell-free ubiquitination assay results. HEK293T cells overexpressing FLAG-IRS-2 or FLAG were serum starved and lysed. Immunoprecipitates adsorbed on anti-FLAG antibody-conjugated beads were subjected to cell-free ubiquitination assay using GST-Nedd4 or GST. (b–e) IRS-2 ubiquitination by Nedd4 overexpression. HEK293 cells (b) or HEK293T cells expressing the indicated proteins (c–e) were serum starved. A portion of the cell lysate was mixed with 2% SDS, boiled for 5 min and diluted. These denatured samples (indicated lanes inband all immunoprecipitates inc–e) and native samples were subjected to immunoprecipitation and immunoblotting as indicated. Inc, purified monoubiquitin was subjected to immunoblotting, to confirm that FK1 antibody does not recognize monoubiquitin (upper panel). UbK0 is an ubiquitin mutant in which all Lys residues were substituted to Arg. Nedd4Y592A/F694Ais a mutant lacking ubiquitin chain-elongation activity. (f) Location of Lys residues in IRS-2. IPK, intermediate region flanking the PTB domain and the KRLB region; KRLB, kinase regulatory loop-binding region; C1-3, C-terminal region 1–3. (g,h) Effects of the indicated Lys-Arg substitution in IRS-2 on its ubiquitination by Need4. HEK293T cells overexpressing indicated proteins were serum starved. Cell lysates were denatured and analysed by immunoprecipitation and immunoblotting as indicated (g). Densitometric analyses were performed. Ubiquitination levels of IRS-2 were normalized to its protein levels, and the means±s.d. of four independent experiments were shown inh. *Significant difference (P<0.05, one-way analysis of variance followed by Tukey–Kramer test). (i) Quantitative MS analysis results. IRS-2 immunoprecipitates derived from HEK293T cells expressing IRS-2 (-Nedd4) or IRS-2 and Nedd4 (+Nedd4) were treated with trypsin and Asp-N. Peptides with ubiquitin remnant motif were enriched and subjected to LC-MS/MS analysis. The graph shows means±s.d. of three independent experiments. *Significant difference from control (P<0.05, Student’st-test). Figure 2: Nedd4 induces IRS-2 monoubiquitination. ( a ) Cell-free ubiquitination assay results. HEK293T cells overexpressing FLAG-IRS-2 or FLAG were serum starved and lysed. Immunoprecipitates adsorbed on anti-FLAG antibody-conjugated beads were subjected to cell-free ubiquitination assay using GST-Nedd4 or GST. ( b – e ) IRS-2 ubiquitination by Nedd4 overexpression. HEK293 cells ( b ) or HEK293T cells expressing the indicated proteins ( c – e ) were serum starved. A portion of the cell lysate was mixed with 2% SDS, boiled for 5 min and diluted. These denatured samples (indicated lanes in b and all immunoprecipitates in c – e ) and native samples were subjected to immunoprecipitation and immunoblotting as indicated. In c , purified monoubiquitin was subjected to immunoblotting, to confirm that FK1 antibody does not recognize monoubiquitin (upper panel). UbK0 is an ubiquitin mutant in which all Lys residues were substituted to Arg. Nedd4 Y592A/F694A is a mutant lacking ubiquitin chain-elongation activity. ( f ) Location of Lys residues in IRS-2. IPK, intermediate region flanking the PTB domain and the KRLB region; KRLB, kinase regulatory loop-binding region; C1-3, C-terminal region 1–3. ( g , h ) Effects of the indicated Lys-Arg substitution in IRS-2 on its ubiquitination by Need4. HEK293T cells overexpressing indicated proteins were serum starved. Cell lysates were denatured and analysed by immunoprecipitation and immunoblotting as indicated ( g ). Densitometric analyses were performed. Ubiquitination levels of IRS-2 were normalized to its protein levels, and the means±s.d. of four independent experiments were shown in h . *Significant difference ( P <0.05, one-way analysis of variance followed by Tukey–Kramer test). ( i ) Quantitative MS analysis results. IRS-2 immunoprecipitates derived from HEK293T cells expressing IRS-2 (-Nedd4) or IRS-2 and Nedd4 (+Nedd4) were treated with trypsin and Asp-N. Peptides with ubiquitin remnant motif were enriched and subjected to LC-MS/MS analysis. The graph shows means±s.d. of three independent experiments. *Significant difference from control ( P <0.05, Student’s t -test). Full size image Two antibodies were used to examine whether Nedd4-induced IRS-2 ubiquitination is monoubiquitination or polyubiquitination. Anti-ubiquitin antibody P4D1 can recognize both monoubiquitin and polyubiquitin chains, whereas FK1 only recognizes polyubiquitin chains [25] . IRS-2 ubiquitination was detected only with P4D1 ( Fig. 2c ). We also compared Nedd4-dependent IRS-2 ubiquitination in cells overexpressing haemagglutinin (HA)-tagged ubiquitin (HA-Ub) or modified HA-Ub in which all Lys residues were replaced with Arg (HA-UbK0). The molecular weight of IRS-2 conjugated with HA-UbK0 was similar to that with HA-Ub ( Fig. 2d ). IRS-2 conjugated with HA-UbK0 was less than that with HA-Ub, possibly due to low expression level of HA-UbK0 in our experimental system. IRS-2 ubiquitination was also detected when cells were overexpressing Nedd4 Y592A or Nedd4 F694A that can conjugate single ubiquitin to substrates but lack ubiquitin chain elongation activity [26] ( Fig. 2e ). Taken together, these results indicated that IRS-2 ubiquitination by Nedd4 occurs as monoubiquitination at single or multiple lysine residues. To map the IRS-2 ubiquitination sites, we generated a series of IRS-2 mutants in which all Lys residues in a defined region are replaced with Arg ( Fig. 2f ). Mutation of all Lys residues in the C1–C3 region (C1–C3 KR) abolished IRS-2 ubiquitination ( Fig. 2g,h ), indicating that IRS-2 ubiquitination sites are located in this region. Mutation in the C3 region largely decreased IRS-2 ubiquitination ( Fig. 2g,h ), indicating that Lys residues in the C3 region are more important. Further analysis using site-directed mutagenesis targeting Lys residues in the C3 region revealed that Lys 1331 is the most frequently ubiquitinated site ( Fig. 2g,h ). In parallel experiments, we used liquid chromatography–tandem mass spectrometry (LC-MS/MS) to identify ubiquitination sites in HEK293T cells overexpressing Nedd4. We detected several IRS-2 peptides containing the ubiquitin remnant motif (K-ɛ-GG) marking ubiquitinated proteins after trypsinolysis ( Supplementary Fig. 3b ). Importantly, the peptide containing Lys 1331 with the ubiquitin remnant was detected ( Supplementary Fig. 3c ). Quantitative MS analysis revealed that the peptide containing Lys 1331 with ubiquitin remnant was intensely increased by Nedd4 overexpression ( Fig. 2I and Supplementary Fig. 3d,e ). IRS-2 monoubiquitination enhances IGF-I signalling We investigated the effects of Nedd4 overexpression on IGF-I signalling in HEK293 cells. Although Nedd4 overexpression did not affect the levels of IGF-IR or IGF-I-induced IGF-IR tyrosine phosphorylation ( Fig. 3a,b and Supplementary Fig. 4a ), it enhanced IGF-I-induced IRS-2 tyrosine phosphorylation and increased the amounts of PI3K bound to IRS-2 ( Fig. 3a,b ). Time-course experiments showed that Nedd4 increased the magnitude of IGF-I-induced IRS-2 tyrosine phosphorylation at 1 and 3 min ( Fig. 3c ). In contrast, Nedd4 overexpression resulted in modest decreases in the total IRS-1 levels and IGF-I-induced IRS-1 tyrosine phosphorylation ( Supplementary Fig. 4b,c ). Nedd4 overexpression did not affect the amounts of PI3K bound to IRS-1 ( Supplementary Fig. 4b ). 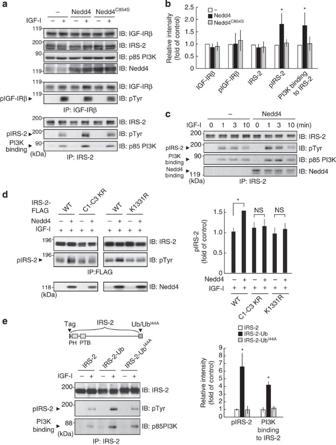Figure 3: Need4 enhances IGF-I signalling by regulating IRS-2 ubiquitination. (a–c) Effects of Nedd4 overexpression on IGF-I signalling. HEK293 cells overexpressing Nedd4 or Nedd4C854S(a ubiquitin ligase inactive mutant) together with IRS-2 were serum starved, followed by IGF-I stimulation (100 ng ml−1) for 1 min (a) or the indicated durations (c). Lysates were subjected to immunoprecipitation and immunoblotting using the indicated antibodies. The results ofawere quantified by densitometric analysis. IGF-I-induced tyrosine phosphorylation levels of IGF-IRβ and IRS-2 were normalized to their protein levels in immunoprecipitates and p85 PI3K bound to IRS-2 was normalized to IRS-2 levels in immunoprecipitates. The means±s.d. of three independent experiments are shown inb. *Significant difference from control (P<0.05, one-way analysis of variance (ANOVA) followed by Tukey–Kramer test). (d,e) Effects of the expression of IRS-2 ubiquitination site mutants (d) and an IRS-2 -ubiquitin chimeric protein (e) on IRS-2 tyrosine phosphorylation. HEK293 cells overexpressing indicated proteins were subjected to experiments similar toa. UbI44A, ubiquitin unable to interact with ubiquitin-binding domains. IGF-I-induced tyrosine phosphorylation levels of IRS-2 and PI3K bound to IRS-2 were normalized to IRS-2 protein levels in immunoprecipitates. Means±s.d. of six (d) or three (e) independent experiments are shown. *Significant difference from control (P<0.05, one-way ANOVA followed by Tukey–Kramer test); NS, not significant. Figure 3: Need4 enhances IGF-I signalling by regulating IRS-2 ubiquitination. ( a – c ) Effects of Nedd4 overexpression on IGF-I signalling. HEK293 cells overexpressing Nedd4 or Nedd4 C854S (a ubiquitin ligase inactive mutant) together with IRS-2 were serum starved, followed by IGF-I stimulation (100 ng ml −1 ) for 1 min ( a ) or the indicated durations ( c ). Lysates were subjected to immunoprecipitation and immunoblotting using the indicated antibodies. The results of a were quantified by densitometric analysis. IGF-I-induced tyrosine phosphorylation levels of IGF-IRβ and IRS-2 were normalized to their protein levels in immunoprecipitates and p85 PI3K bound to IRS-2 was normalized to IRS-2 levels in immunoprecipitates. The means±s.d. of three independent experiments are shown in b . *Significant difference from control ( P <0.05, one-way analysis of variance (ANOVA) followed by Tukey–Kramer test). ( d , e ) Effects of the expression of IRS-2 ubiquitination site mutants ( d ) and an IRS-2 -ubiquitin chimeric protein ( e ) on IRS-2 tyrosine phosphorylation. HEK293 cells overexpressing indicated proteins were subjected to experiments similar to a . Ub I44A , ubiquitin unable to interact with ubiquitin-binding domains. IGF-I-induced tyrosine phosphorylation levels of IRS-2 and PI3K bound to IRS-2 were normalized to IRS-2 protein levels in immunoprecipitates. Means±s.d. of six ( d ) or three ( e ) independent experiments are shown. *Significant difference from control ( P <0.05, one-way ANOVA followed by Tukey–Kramer test); NS, not significant. Full size image We next investigated the underlying mechanism. In mouse embryonic fibroblasts, Nedd4 was reported to maintain cell-surface IGF-IR levels by suppressing the abundance of the adaptor protein Grb10 (ref. 16 ). However, Nedd4 overexpression neither affected cell-surface IGF-IR levels nor Grb10 levels in HEK293 cells ( Supplementary Fig. 4c,d ). The Nedd4-induced increase in IRS-2 tyrosine phosphorylation was reduced by the deletion of the Nedd4 amino-terminal region (IRS-2-binding region; Supplementary Fig. 4e ) and was abolished by the substitution of Nedd4 Cys 854 with Ser, which inactivates Nedd4 ubiquitin ligase activity [14] ( Fig. 3a,b ). These results suggest that the Nedd4-induced IRS-2 ubiquitination leads to the enhancement of IRS-2 tyrosine phosphorylation. To elucidate whether monoubiquitination of IRS-2 is required for the increased IGF signalling, we used several IRS-2 ubiquitination site mutants. Both IRS-2 C1-C3 KR mutation and K1331R mutation suppressed Nedd4-dependent increases in IRS-2 tyrosine phosphorylation ( Fig. 3d ), indicating that monoubiquitination at IRS-2 Lys 1331 is required for Nedd4-induced enhancement of IRS-2 tyrosine phosphorylation. As Lys 1331 is near the IRS-2 carboxy terminus ( Fig. 2f ), we also generated IRS-2 fused with monoubiquitin at the C terminus. When cells overexpressing this chimeric protein were stimulated with IGF-I, it was tyrosine phosphorylated and bound to PI3K more intensely than intact IRS-2 ( Fig. 3e ). Therefore, fusion of a single ubiquitin molecule to IRS-2 is sufficient to enhance its tyrosine phosphorylation in response to IGF-I. Ubiquitin is recognized by a number of ubiquitin-binding proteins. These proteins target the ubiquitinated proteins to proteasome, sorting machinery or de-ubiquitinating enzymes [27] . Ile 44 of ubiquitin has been shown to be crucial for its interaction with ubiquitin-binding proteins [27] . When the Ile 44 in the IRS-2-ubiquitin chimeric protein was substituted to Ala, Nedd4-dependent increases in IRS-2 tyrosine phosphorylation was suppressed ( Fig. 3e ), suggesting that recognition of IRS-2 by ubiquitin-binding protein(s) is required for the Nedd4-dependent increases in IRS-2 tyrosine phosphorylation. Epsin1 mediates the Nedd4 effects on IGF-I signalling To identify proteins that recognize ubiquitinated IRS-2, we studied several ubiquitin-binding proteins in the endocytosis machinery, including Eps15, Eps15R, Epsin1, HRS and TSG101 (ref. 28 ). Among them, the association of Epsin1 with IRS-2 was increased by overexpression of Nedd4 ( Fig. 4a ) and the IRS-2-ubiquitin chimeric protein ( Supplementary Fig. 5a ). Nedd4 overexpression did not affect the association of the other ubiquitin-binding proteins with IRS-2 ( Supplementary Fig. 5b ). The association of IRS-2 with Epsin1 was suppressed by the mutation of IRS-2 ubiquitination sites ( Fig. 4b ) and by the deletion of Epsin1 ubiquitin-interacting motifs (UIMs) [29] ( Fig. 4b and Supplementary Fig. 5c ). These results indicate that Epsin1 UIMs bind to the ubiquitin conjugated on IRS-2. Further analysis revealed that Epsin1 knockdown suppressed the effect of Nedd4 overexpression on IRS-2 tyrosine phosphorylation, while it had no effect on IGF-IR tyrosine phosphorylation ( Fig. 4c ). These results indicate that ubiquitinated IRS-2 is bound to Epsin1 and this molecular interaction is required for the enhanced IRS-2 tyrosine phosphorylation in response to IGF-I. 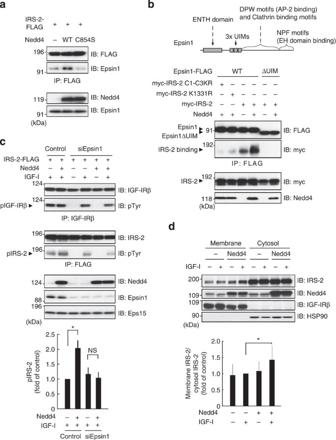Figure 4: Epsin1 mediates the Nedd4 effect on IGF-I signalling. (a) Effects of Nedd4 overexpression on the IRS-2 and Epsin1 interaction. HEK293T cells overexpressing indicated proteins were serum starved. Lysates were subjected to immunoprecipitation and immunoblotting as indicated. (b) Effects of IRS-2 ubiquitination site mutation or deletion of Epsin1 UIM motif. Epsin1 structure is shown in the upper panel. ENTH, Epsin N-terminal homology; UIM, ubiquitin-interacting motif; DPW, Asp-Pro-Trp; AP-2, adaptor protein-2; NPF, Asn-Pro-Phe; EH, Eps15 homology. HEK293T cells overexpressing indicated proteins were serum starved. Lysates were subjected to immunoprecipitation and immunoblotting as indicated. (c) Role of Epsin1 in IGF-I-induced IRS-2 tyrosine phosphorylation. HEK293 cells transfected with indicated plasmids and/or siRNAs were serum starved and then treated with 100 ng ml−1IGF-I for 1 min. Cell lysates were subjected to immunoprecipitation and immunoblotting. Densitometric analyses of cells with IGF-I stimulation were performed and tyrosine phosphorylation levels of IRS-2 were normalized to IRS-2 protein levels in immunoprecipitates. The means±s.d. of three independent experiments are shown in the graph. *Significant difference (P<0.05, one-way analysis of variance (ANOVA) followed by Tukey–Kramer test). (d) Regulation of IRS-2 subcellular localization by Nedd4. HEK293 cells overexpressing Nedd4 and IRS-2 were serum starved, followed by IGF-I stimulation (100 ng ml−1, 1 min). Cell lysates were fractionated into membrane/cytosol fractions, followed by immunoblotting using the indicated antibodies. Densitometric analyses were performed and the ratio of IRS-2 in the membrane fraction to IRS-2 in the cytosol fraction was calculated. The graph shows the mean±s.d. of the densitometric analysis of six independent experiments. *Significant difference (P<0.05, one-way ANOVA followed by Tukey–Kramer test). Figure 4: Epsin1 mediates the Nedd4 effect on IGF-I signalling. ( a ) Effects of Nedd4 overexpression on the IRS-2 and Epsin1 interaction. HEK293T cells overexpressing indicated proteins were serum starved. Lysates were subjected to immunoprecipitation and immunoblotting as indicated. ( b ) Effects of IRS-2 ubiquitination site mutation or deletion of Epsin1 UIM motif. Epsin1 structure is shown in the upper panel. ENTH, Epsin N-terminal homology; UIM, ubiquitin-interacting motif; DPW, Asp-Pro-Trp; AP-2, adaptor protein-2; NPF, Asn-Pro-Phe; EH, Eps15 homology. HEK293T cells overexpressing indicated proteins were serum starved. Lysates were subjected to immunoprecipitation and immunoblotting as indicated. ( c ) Role of Epsin1 in IGF-I-induced IRS-2 tyrosine phosphorylation. HEK293 cells transfected with indicated plasmids and/or siRNAs were serum starved and then treated with 100 ng ml −1 IGF-I for 1 min. Cell lysates were subjected to immunoprecipitation and immunoblotting. Densitometric analyses of cells with IGF-I stimulation were performed and tyrosine phosphorylation levels of IRS-2 were normalized to IRS-2 protein levels in immunoprecipitates. The means±s.d. of three independent experiments are shown in the graph. *Significant difference ( P <0.05, one-way analysis of variance (ANOVA) followed by Tukey–Kramer test). ( d ) Regulation of IRS-2 subcellular localization by Nedd4. HEK293 cells overexpressing Nedd4 and IRS-2 were serum starved, followed by IGF-I stimulation (100 ng ml −1 , 1 min). Cell lysates were fractionated into membrane/cytosol fractions, followed by immunoblotting using the indicated antibodies. Densitometric analyses were performed and the ratio of IRS-2 in the membrane fraction to IRS-2 in the cytosol fraction was calculated. The graph shows the mean±s.d. of the densitometric analysis of six independent experiments. *Significant difference ( P <0.05, one-way ANOVA followed by Tukey–Kramer test). Full size image Epsin1 is localized at the plasma membrane, especially at sites where clathrin-coated pits will be formed [30] . Subcellular fractionation analysis showed that Nedd4 overexpression increased IRS-2 levels in the membrane fraction when cells were stimulated with IGF-I ( Fig. 4d ). These data suggested that Nedd4 recruits IRS-2 to the plasma membrane, where IRS-2 is effectively phosphorylated by the IGF-IR tyrosine kinase. Nedd4 enhances IGF-I signalling in thyrocytes Prolonged pretreatment of nontransformed thyroid FRTL-5 cells with TSH or other cAMP-generating reagents is known to enhance IGF-I-dependent IRS-2 tyrosine phosphorylation and DNA synthesis [10] , [22] , [23] . As shown in Fig. 5a and Supplementary Fig. 6a , dibutyryl cAMP treatment of FRTL-5 cells increased the association of endogenous Nedd4 with IRS-2. Pull-down analysis using GST-IRS-2 (aa 1–329) or GST-Nedd4 (aa 1–226) showed that cAMP treatment increases the affinity of Nedd4 for IRS-2 ( Fig. 5b ). In comparison, no association of IRS-2 with Nedd4-2 was detected ( Fig. 5a ). It should be noted that cAMP treatment changed the IRS-2 electrophoretic mobility ( Fig. 5a and subsequent figures). Our previous study showed that cAMP treatment does not change IRS-2 levels and the cAMP treatment-induced IRS-2 mobility shift is due to its Ser/Thr phosphorylation [10] . Although Nedd4 was reported to interact with IGF-IR previously in other cell types [15] , our analysis indicated that IGF-IR was not co-immunoprecipitated with IRS-2 ( Supplementary Fig. 6b ), indicating that Nedd4 associates with IGF-IR and IRS-2, independently. Next, we tested the effects of cAMP treatment on IRS-2 ubiquitination. Immunoblotting analysis with P4D1 and FK1 revealed that cAMP treatment increased monoubiquitination of IRS-2 ( Fig. 5c ). Subcellular fractionation showed that cAMP treatment markedly increased the amounts of IRS-2 in the membrane fraction ( Fig. 5d ). 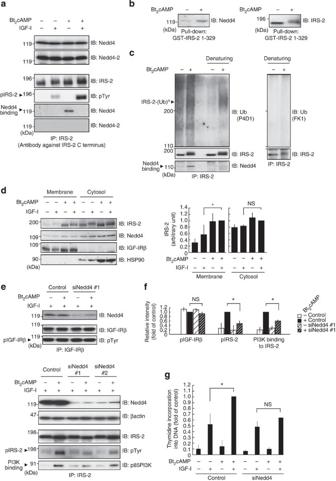Figure 5: Nedd4 enhances IGF-I signalling in thyrocytes. In the experiments described below, FRTL-5 cells were treated with or without 1 mM dibutyryl cAMP for 24 h. In samples indicated ‘+IGF-I’, cells were then stimulated with 100 ng ml−1IGF-I for 1 min (a,d,e) or 24 h (g) after cAMP treatment. *Significant difference (P<0.05). (a) Effects of cAMP treatment on the Nedd4 and IRS-2 complex formation. Cell lysates were subjected to immunoprecipitation and immunoblotting as indicated. (b) Effects of cAMP treatment on the Nedd4 and IRS-2 binding in cell-free binding assay. Cell lysates were subjected to pull-down analysis using indicated GST-fused proteins. (c) Effects of cAMP treatment on IRS-2 ubiquitination. Native samples and denatured samples were subjected to immunoprecipitation and immunoblotting as indicated. (d) Effects of cAMP and/or IGF-I treatments on IRS-2 subcellular localization. Cell lysates were fractionated into membrane/cytosol fractions, followed by immunoblotting. Right panel shows the densitometric analysis results. Mean±s.d. of three independent experiments. *Significant difference (P<0.05, one-way analysis of variance (ANOVA) followed by Tukey–Kramer test). (e–g) Effect of Nedd4 knockdown on IGF-I signalling and IGF-I-induced DNA synthesis. Cells transfected with Nedd4 siRNAs were treated with dibutyryl cAMP followed by IGF-I stimulation. Lysates were subjected to immunoprecipitation and immunoblotting (e). Densitometric analyses were performed. Tyrosine phosphorylation levels of IGF-IRβ and IRS-2 were normalized to their protein levels in immunoprecipitates and p85 PI3K bound to IRS-2 was normalized to IRS-2 levels in immunoprecipitates. Means±s.d. of seven independent experiments are shown inf. [3H]thymidine incorporation into DNA during 20–24 h of IGF-I treatment time was measured. The values were normalized and the means±s.d. of three independent experiments are shown ing. *Significant difference (P<0.05, one-way ANOVA followed by Tukey–Kramer test). Figure 5: Nedd4 enhances IGF-I signalling in thyrocytes. In the experiments described below, FRTL-5 cells were treated with or without 1 mM dibutyryl cAMP for 24 h. In samples indicated ‘+IGF-I’, cells were then stimulated with 100 ng ml −1 IGF-I for 1 min ( a , d , e ) or 24 h ( g ) after cAMP treatment. *Significant difference ( P <0.05). ( a ) Effects of cAMP treatment on the Nedd4 and IRS-2 complex formation. Cell lysates were subjected to immunoprecipitation and immunoblotting as indicated. ( b ) Effects of cAMP treatment on the Nedd4 and IRS-2 binding in cell-free binding assay. Cell lysates were subjected to pull-down analysis using indicated GST-fused proteins. ( c ) Effects of cAMP treatment on IRS-2 ubiquitination. Native samples and denatured samples were subjected to immunoprecipitation and immunoblotting as indicated. ( d ) Effects of cAMP and/or IGF-I treatments on IRS-2 subcellular localization. Cell lysates were fractionated into membrane/cytosol fractions, followed by immunoblotting. Right panel shows the densitometric analysis results. Mean±s.d. of three independent experiments. *Significant difference ( P <0.05, one-way analysis of variance (ANOVA) followed by Tukey–Kramer test). ( e – g ) Effect of Nedd4 knockdown on IGF-I signalling and IGF-I-induced DNA synthesis. Cells transfected with Nedd4 siRNAs were treated with dibutyryl cAMP followed by IGF-I stimulation. Lysates were subjected to immunoprecipitation and immunoblotting ( e ). Densitometric analyses were performed. Tyrosine phosphorylation levels of IGF-IRβ and IRS-2 were normalized to their protein levels in immunoprecipitates and p85 PI3K bound to IRS-2 was normalized to IRS-2 levels in immunoprecipitates. Means±s.d. of seven independent experiments are shown in f . [ 3 H]thymidine incorporation into DNA during 20–24 h of IGF-I treatment time was measured. The values were normalized and the means±s.d. of three independent experiments are shown in g . *Significant difference ( P <0.05, one-way ANOVA followed by Tukey–Kramer test). Full size image We then studied the role of Nedd4 in IGF-I signalling and mitogenic activity in FRTL-5 cells. Nedd4 knockdown neither affected IGF-I-induced IGF-IR tyrosine phosphorylation ( Fig. 5e,f ) nor Grb10 levels ( Supplementary Fig. 6c ). cAMP pretreatment enhanced IGF-I-induced IRS-2 tyrosine phosphorylation and this was suppressed by Nedd4 knockdown ( Fig. 5e,f ) but not by Nedd4-2 knockdown ( Supplementary Fig. 6d ). cAMP pretreatment enhanced IGF-I-induced DNA synthesis and this was abolished by Nedd4 knockdown ( Fig. 5g ). These data indicated that Nedd4 is required for cAMP-dependent enhancement of IGF-I signalling and mitogenic activity. Nedd4 enhances IGF-I signalling in prostate cancer cells We also investigated the possible role of Nedd4 in IGF-I action in prostate cancer cells. We confirmed that Nedd4 associated with IRS-2 in prostate cancer DU145 cells and PC-3 cells ( Fig. 6a ). Nedd4 knockdown did not affect IGF-I-induced IGF-IR tyrosine phosphorylation in PC-3 cells, whereas it decreased IRS-2 tyrosine phosphorylation and the amounts of PI3K bound to IRS-2 ( Fig. 6b ). Nedd4-2 was not detected in these cells ( Supplementary Fig. 7 ). Epsin1 knockdown also decreased IGF-I-induced IRS-2 tyrosine phosphorylation ( Fig. 6c ), supporting our conclusion that Epsin1 mediates Nedd4-induced enhancement of IGF-I signalling. 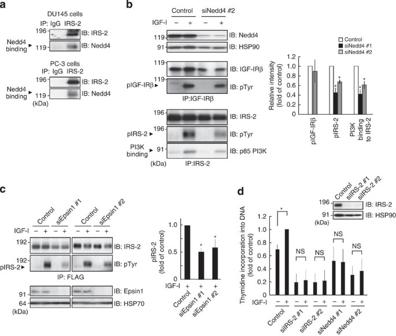Figure 6: Nedd4 enhances IGF-I signalling in prostate cancer cells. (a) The association of Nedd4 with IRS-2. DU145 cells or PC-3 cells were serum starved and cell lysates were subjected to immunoprecipitation and immunoblotting as indicated. (b,c) Effects of knockdown of Nedd4 or Epsin1 on IGF-I signalling in PC-3 cells. Cells transfected with indicated siRNAs were serum starved and then treated with or without 100 ng ml−1IGF-I for 1 min. Lysates were subjected to immunoprecipitation and immunoblotting as shown. Densitometric analyses of samples with IGF-I stimulation were performed. Tyrosine phosphorylation levels of IGF-IRβ and IRS-2 were normalized to their protein levels in immunoprecipitates. p85 PI3K bound to IRS-2 was normalized to IRS-2 levels in immunoprecipitates. Means±s.d. of three to five independent experiments are shown in the right panel. *Significant difference from control (P<0.05, one-way analysis of variance (ANOVA) followed by Tukey–Kramer test). (d) Effects of knockdown of IRS-2 or Nedd4 on IGF-I-induced DNA synthesis in PC-3 cells. Cells transfected with IRS-2 siRNAs or Nedd4 siRNAs were serum starved for 48 h and then treated with or without 100 ng ml−1IGF-I for 16 h. [3H]thymidine incorporation into DNA during 13–16 h of IGF-I treatment time was measured. The values were normalized and the means±s.d. of three independent experiments are shown. Right insert shows the immunoblotting results. *Significant difference (P<0.05, one-way ANOVA followed by Tukey–Kramer test). Figure 6: Nedd4 enhances IGF-I signalling in prostate cancer cells. ( a ) The association of Nedd4 with IRS-2. DU145 cells or PC-3 cells were serum starved and cell lysates were subjected to immunoprecipitation and immunoblotting as indicated. ( b , c ) Effects of knockdown of Nedd4 or Epsin1 on IGF-I signalling in PC-3 cells. Cells transfected with indicated siRNAs were serum starved and then treated with or without 100 ng ml −1 IGF-I for 1 min. Lysates were subjected to immunoprecipitation and immunoblotting as shown. Densitometric analyses of samples with IGF-I stimulation were performed. Tyrosine phosphorylation levels of IGF-IRβ and IRS-2 were normalized to their protein levels in immunoprecipitates. p85 PI3K bound to IRS-2 was normalized to IRS-2 levels in immunoprecipitates. Means±s.d. of three to five independent experiments are shown in the right panel. *Significant difference from control ( P <0.05, one-way analysis of variance (ANOVA) followed by Tukey–Kramer test). ( d ) Effects of knockdown of IRS-2 or Nedd4 on IGF-I-induced DNA synthesis in PC-3 cells. Cells transfected with IRS-2 siRNAs or Nedd4 siRNAs were serum starved for 48 h and then treated with or without 100 ng ml −1 IGF-I for 16 h. [ 3 H]thymidine incorporation into DNA during 13–16 h of IGF-I treatment time was measured. The values were normalized and the means±s.d. of three independent experiments are shown. Right insert shows the immunoblotting results. *Significant difference ( P <0.05, one-way ANOVA followed by Tukey–Kramer test). Full size image Cultured PC-3 cells secrete IGF-I and -II into media, which stimulates their proliferation [31] , [32] . We observed that IGF-I stimulation increased DNA synthesis in PC-3 cells and this was decreased below the basal levels by Nedd4 knockdown as well as by IRS-2 knockdown ( Fig. 6d ), indicating that both Nedd4 and IRS-2 are necessary for their proliferation in response to endogenously secreted IGFs and exogenously added IGF-I. Together, these data indicate the requirement of the Nedd4-IRS-2 complex for maximum IGF-I signalling as well as mitogenic activity in PC-3 cells. Nedd4 accelerates zebrafish embryonic growth through IRS-2 To elucidate Nedd4 functions in an in vivo setting, we used the zebrafish embryo model. The IGF signalling pathway is highly conserved and previous studies suggest that IGFs regulate zebrafish embryonic growth by promoting cell proliferation and survival, without changing developmental patterning [33] , [34] . As shown in Fig. 7a–c , Nedd4 overexpression increased zebrafish embryo growth (body length) and developmental timing (somite number) without major organ loss or patterning abnormalities. These biological actions of Nedd4 were abolished by knocking down Irs2, using morpholino antisense oligos (MO) ( Fig. 7a–c ). Specific translation block with Irs2 MO and Nedd4 overexpression were confirmed ( Supplementary Fig. 8a-c ). Taken together, these data indicate that Nedd4 accelerates zebrafish embryonic growth through Irs2. 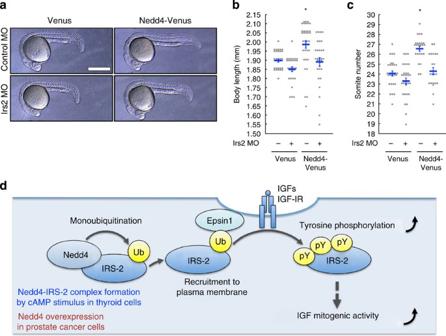Figure 7: Nedd4 accelerates zebrafish embryonic growth through Irs-2. (a) Nedd4-Venus mRNA or Venus mRNA was co-injected with either Irs2 MO or control MO into one- to two-cell stage zebrafish embryos. The embryos were raised to 22 h post fertilization and representative embryos are shown. Scale bar, 500 μm. (b,c) Values of body length and somite number are plotted. Blue lines indicate the means±s.e.m. (n=21–34). *Significant difference from the control group (P<0.05, one-way analysis of variance followed by Tukey–Kramer test). (d) Working model on how Nedd4 enhances IGF signalling and mitogenic activity (a detailed explanation is given in the Discussion). Figure 7: Nedd4 accelerates zebrafish embryonic growth through Irs-2. ( a ) Nedd4-Venus mRNA or Venus mRNA was co-injected with either Irs2 MO or control MO into one- to two-cell stage zebrafish embryos. The embryos were raised to 22 h post fertilization and representative embryos are shown. Scale bar, 500 μm. ( b , c ) Values of body length and somite number are plotted. Blue lines indicate the means±s.e.m. ( n =21–34). *Significant difference from the control group ( P <0.05, one-way analysis of variance followed by Tukey–Kramer test). ( d ) Working model on how Nedd4 enhances IGF signalling and mitogenic activity (a detailed explanation is given in the Discussion). Full size image In this study, we identified Nedd4 as a novel IRS-2-associated protein and elucidated the molecular mechanisms of the complex formation, IRS-2 ubiquitination and role of this interaction in IGF action in normal and cancer cells in vitro , as well as in zebrafish embryos in vivo . Wiesner et al. [24] suggested that the Nedd4 C2 domain binds to its HECT domain and this intramolecular binding inhibits its ubiquitin ligase activity. In this study, we discovered that IRS-2 and the Nedd4 HECT domain competitively bind to the C2 domain. IRS-2 binds to the Nedd4 C2 domain in a region overlapping with the HECT-binding site. Thus, we speculate that the dissociation of the C2 and HECT domains not only restores Nedd4 ligase activity but also opens up a substrate-binding site, which enables its recognition of some substrates, including IRS-2. It cannot be ruled out that other factor(s) mediate Nedd4–IRS-2 interaction. Crystal structure analysis will aid in understanding the molecular basis of the regulation of this complex formation. This study demonstrates that Nedd4 induces monoubiquitination at single or multiple Lys residues in the IRS-2 C-terminal region. Ubiquitinated IRS-2 in FRTL-5 cells showed a little higher molecular weight than that in HEK293 cells ( Figs 2b and 5c ), indicating a different number of monoubiquitinated lysine residues. Nedd4 conjugated more ubiquitin molecules to IRS-2 in a cell-free system than in cells ( Fig. 2a ). Some ubiquitin molecules may be removed from IRS-2 by de-ubiquitination enzymes in cells. In fact, we observed significant levels of de-ubiquitination enzyme USP7 associated with IRS-2 in HEK293 cells [35] . Further analysis is needed to elucidate how Nedd4 induces monoubiquitination of IRS-2. Several ubiquitin ligases other than Nedd4 have been shown to ubiquitinate IRS-1/2, but they all induce proteasomal degradation of IRS-1/2 and suppress IGF/insulin signalling [36] , [37] , [38] , [39] . In contrast, we demonstrated that Nedd4 enhances IGF-I signalling in this study, indicating a unique role for Nedd4 in IGF signal regulation. Conjugation of polyubiquitin chains consisting of four or more ubiquitin molecules to substrate proteins is required for their proteasomal degradation [40] , which can explain why Nedd4 does not induce IRS-2 degradation. Our data suggest that Nedd4 increases the association of IRS-2 with Epsin1 and this in turn promotes the translocation of IRS-2 from the cytosol to the plasma membrane. Epsin1 UIMs mediate the association of ubiquitinated IRS-2 with Epsin1. Epsin1 is localized to the plasma membrane and facilitates the formation of clathrin-coated invaginations through its other domains and motifs (schematically represented in Fig. 4b ) [30] , [41] . We speculate that Epsin1 may recruit the ubiquitinated IRS-2 to the position adjacent to the plasma membrane through physical interaction. As IGF-IR internalizes through the clathrin-dependent pathway [42] , it is attractive to postulate that Nedd4 may induce the co-localization of IRS-2 and IGF-IR at a specific plasma membrane compartment, where high levels of Epsin1 are present and clathrin-coated pits are forming. Their co-localization facilitates phosphorylation of IRS-2 by the IGF-IR tyrosine kinase. This model is strongly supported by our result that Epsin1 knockdown suppressed the effect of Nedd4 on IRS-2 tyrosine phosphorylation ( Fig. 4c ). It is unclear why different IGF-I-dependency of IRS-2 translocation was shown in subcellular fractionation of HEK293 cells and FRTL-5 cells ( Figs 4d and 5d ). Further studies are needed to elucidate molecular mechanisms underlying Epsin1-mediated modulation of IGF-I signalling. Thyroid epithelial cells synergistically proliferate in response to IGF-I and TSH in vitro [43] , [44] , [45] , which is thought to be important for thyroid morphogenesis and thyroid hormone homeostasis [46] . We previously reported that TSH or other cAMP-generating reagents enhance IGF-I-induced cell proliferation in thyroid FRTL-5 cells [44] . In this study, we showed that cAMP stimulus induces the association of Nedd4 with IRS-2, IRS-2 monoubiquitination and recruitment of IRS-2 to the membrane fraction. Nedd4 is required for the cAMP-dependent enhancement of IRS-2 tyrosine phosphorylation and DNA synthesis induced by IGF-I. We conclude that cAMP stimulus triggers the mechanisms by which Nedd4 enhances IRS-2-mediated signalling. In various endocrine tissues, IGFs and tropic hormones synergistically regulate cell proliferation, differentiation and hormone synthesis [6] . As tropic hormones generally use the cAMP pathway, we speculate that Nedd4 may play roles in the cross-talk between IGFs and other hormones. In this study, we also detected the Nedd4–IRS-2 complex in prostate cancer cells. Nedd4 knockdown suppressed IGF-I-induced IRS-2 tyrosine phosphorylation and DNA synthesis, suggesting that Nedd4 enhances IRS-2-mediated signalling and IGF-I mitogenic activity. It has been reported that Nedd4 promotes prostate cancer development through the ubiquitination and degradation of phosphatase and tensin homologue (PTEN) [17] . However, PC-3 cells are deficient in PTEN [47] , excluding the possibility that the effects of Nedd4 are mediated by the regulation of PTEN in our experiments. The Nedd4-IRS-2 binding may represent a novel drug target at least in prostate cancer. Accumulating evidence suggests that Nedd4 is overexpressed in various cancers and functions as a tumour-promoting factor [17] , [18] , [19] , [20] , [21] . It is important to investigate the contribution of the Nedd4-IRS-2 complex to the development of various cancers. The results of this study show that Nedd4 accelerates zebrafish embryonic growth through Irs2. In mice, Nedd4 deficiency causes delayed embryonic growth [16] . In both cases, Nedd4 modulates embryonic growth without major developmental abnormality of any specific organs. Given that IGF signalling deficiency in various species causes growth retardation without patterning abnormalities [2] , [3] , [4] , [33] , these results imply that Nedd4 is an evolutionarily conserved factor that plays a positive role in embryonic growth, possibly through modulating IGF-IR-IRS-2 signalling activities. It has been reported that Nedd4 acts on multiple IGF signal transducers. As described above, in mouse embryonic fibroblasts, Nedd4 is required to maintain the cell-surface IGF-IR levels [16] . In contrast, others reported that Nedd4 induces degradation of IGF-IR [15] , [48] , [49] . A recent report suggested that Nedd4 may enhance IGF-I-induced IRS-1 tyrosine phosphorylation by antagonizing PTEN, which functions as a tyrosine phosphatase for IRS-1 (ref. 50 ). Nedd4 has also been reported to regulate the stability and subcellular localization of Akt and PTEN [17] , [51] , [52] . In our study, Nedd4 affected neither total nor cell-surface IGF-IR levels, and had little effect on the signalling downstream of IRS-1. These discrepancies may be due to different experimental conditions or cellular models used. It is also possible that these multiple sites of Nedd4 action allow the fine-tuning of IGF signalling in a context-dependent manner. In conclusion, our study demonstrated that Nedd4 enhances IGF-I signalling and mitogenic activity through a novel mechanism ( Fig. 7d ). Nedd4 associates with IRS-2 and conjugates monoubiquitin to IRS-2. Ubiquitinated IRS-2 is in turn recognized by Epsin1, which possibly recruits IRS-2 to the plasma membrane. Consequently, Nedd4 enhances IGF-I-induced tyrosine phosphorylation of IRS-2 by the IGF-IR kinase, which leads to the augmentation of IGF-I signalling and mitogenic activity. Materials Recombinant human IGF-I was kindly donated by Dr Toshiaki Ohkuma (Fujisawa Pharmaceutical Co., Osaka, current Astellas Pharma Inc., Tokyo, Japan). Several anti-IRS-2 antibodies were used in this study. One was obtained from Santa Cruz Biotechnology (sc-8299, Santa Cruz, CA, USA) and another was a home-made antibody against the IRS-2 C-terminal peptide [12] (used in Fig. 5a and Supplementary Fig. 1a,c ). The other anti-IRS-2 antibody against aa 976–1094 (used in Supplementary Fig. 6a , 06-506) was purchased from Millipore (Billerica, MA, USA). Anti-Nedd4 antibody (07-049), anti-p85 PI3K antibody (06-195) and anti-HRS antibody (ABC35) were obtained from Millipore. Anti-myc antibody (clone 9E10, sc-40), anti-ubiquitin antibody (clone P4D1, sc-8017), anti-IGF-IR antibody (sc-713), anti-Grb10 antibody (sc-1026), anti-Eps15 antibody (sc-534), anti-Epsin1 antibody (sc-25521), anti-HSP90 antibody (sc-13119) and horseradish peroxidase (HRP)-linked anti-mouse IgM antibody (sc-2064) were obtained from Santa Cruz Biotechnology. Anti-Eps15R antibody (EP1146Y), anti-TSG101 antibody (EPR7131B) and anti-HSP70 antibody (EP1007Y) were obtained from Abcam (Cambridge, UK). Anti-Nedd4-2 antibody (4013) and anti-ubiquitin remnant motif antibody-conjugated beads were purchased from Cell Signaling (Danvers, MA, USA), and anti-ubiquitin antibody (clone FK1) was from Nippon Bio-Test Laboratories (Tokyo, Japan). Anti-phosphotyrosine antibody (clone PY20), anti-FLAG antibody (clone M2), anti-FLAG M2 antibody-conjugated agarose beads and rabbit IgG were purchased from Sigma-Aldrich (St Louis, MO, USA). Anti-HA antibody (clone 3F10) was from Roche (Basel, Schweiz). HRP-linked anti-mouse IgG antibody (NA931) and HRP-linked anti-rabbit IgG antibody (NA934) were purchased from GE Healthcare (Buckinghamshire, UK). Smal interfering RNAs (siRNAs; 21-mer, having overhanging dTdT at the 3′ terminus) were designed as follows: human IRS-2 #1, 5′-UCGGCUUCGUGAAGCUCAAdTdT-3′, #2, 5′-GGCUGAGCCUCAUGGAGCAdTdT-3′; human Nedd4 #1, 5′-GCAAAUGGCUGCUUUUAAAdTdT-3′, #2, 5′-CCAUGAAUCUAGAAGAACAdTdT-3′; rat Nedd4 #1, 5′-CCAUGAGUCUAGAACAACAdTdT-3′, #2, 5′-GAAGCAGACUGACAUUCCAdTdT-3′; rat Nedd4-2, 5′-GAUCACUUAUCCUAUUUCAdTdT-3′; human Epsin1 #1, 5′-CCAGCUCCGUCUCAGUCCUdTdT-3′; #2, 5′-GCUCCCUCAUGUCAGAGAUdTdT-3′. These siRNAs and a universal negative control RNA were synthesized by Nippon EGT (Toyama, Japan). Rat IRS-1 complementary DNA and human IRS-2 cDNA were prepared as described elsewhere [53] . Mouse Nedd4 cDNA was kindly donated by Dr Sharad Kumar (Queensland University of Technology, Brisbane, Australia.). Mouse Nedd4-2 cDNA was amplified by PCR from mouse brain cDNA library. Ubiquitin cDNA was kindly provided by Dr Takeshi Imamura (Japanese Foundation for Cancer Research, Tokyo, Japan). Rat Epsin1 cDNA and human USP15 cDNA were amplified by PCR from H4IIE hepatocyte cDNA library and Huh7 hepatocyte cDNA library, respectively. Partial zebrafish Irs2 cDNA (NM_200315) was amplified by PCR from zebrafish embryo cDNA library. It contains 5′-untranslated region (UTR) and translation start site of Irs2. cDNAs with deletion or site-directed mutation were generated by standard restriction enzyme- or PCR-based methods. For the construction of expression plasmids, these cDNAs were subcloned into the following vectors; pGEX (GE Healthcare) for the expression of N-terminal glutathione (GST)-tagged protein; modified pEGFP-N1 (Clontech, Mountain View, CA, USA) in which green fluorescent protein gene between the BamHI and NotI sites had been removed, for the expression of intact protein; pFLAG-CMV2 (Sigma-Aldrich) for N-terminal FLAG-tagged protein; pmyc-CMV5 (gift from Dr Jun Nakae, Keio University, Tokyo, Japan) for N-terminal myc-tagged protein; pmyc-CMV5-FLAG that we had generated by inserting FLAG peptide sequence into SalI site, for protein with N-terminal myc-tag and C-terminal FLAG tag; pRKHA for N-terminal HA-tagged protein; pCS2-Venus that was used as template for capped messenger RNA synthesis. Using these vectors, we made Escherichia coli expression plasmids for GST-IRS-2 (aa 1–329) and GST-Nedd4 (wild type; aa 1–226; 1–551; 227–551; 227–887; 552–887; deletion of 227–551 (Δ227–551); Δ251–280, 407–436 and 462–491 (ΔWW)). We also made mammalian expression plasmids for intact IRS-2, FLAG-IRS-2 (wild type; aa 1–545; 1–329; 1–134; 137–329; 137–1338; 330–1338), FLAG-IRS-2-Ub (in which C-terminal di-Gly of ubiquitin was deleted (ΔGG) to prevent its cross-linking to other proteins by ubiquitin ligases), FLAG-IRS-2-Ub I44A (ubiquitin is ΔGG-type), myc-IRS-2-FLAG (wild type and a series of mutants in which indicated Lys residues were substituted to Arg), myc-IRS-2 (wild type, C1-C3 KR and K1331R), myc-IRS-2-Ub (ubiquitin is ΔGG-type), myc-IRS-2-Ub I44A (ubiquitin is ΔGG-type), myc-Nedd4 (wild type; aa 1–551, 503–887 C854S; 552–887 E541A, C854S; I95A, L96A; S126A, L127A; E541A; Y592A; F694A; C854S), FLAG-Nedd4 (wild type; aa 1–502; 1–502 I95A, L96A; 1–502 S126A, L127A), FLAG-Nedd4-2, HA-ubiquitin (HA-Ub), HA-UbK0 (in which all Lys residues were substituted to Arg for prevention of polyubiquitin chain formation), Epsin1-FLAG (wild type; Δ136-256 (ΔUIM)), FLAG-IRS-1 and myc-IRS-1-FLAG. IGF-IR-FLAG plasmid was kindly provided by Dr Iwaki (Osaka University, Osaka, Japan). For the protein expression in zebrafish embryo, Nedd4-Venus plasmids and 5′-UTR Irs2 -Venus plasmids were generated as template for capped RNA synthesis. RNA sequence of 5′-UTR Irs2 -Venus plasmids is shown in Supplementary Fig. 8a . The Irs2 MO (5′-CCATACTTGCGTTGACAGTTTATTT-3′) targeting the translational start site of zebrafish Irs2 mRNA (NM_200315) and the control MO (5′-CCTCTTACCTCAGTTACAATTTATA-3′) were synthesized by Gene Tools, LLC (Philomath, OR, USA). Other chemicals were of the reagent grade available commercially. Cell culture and transfection HEK293 cells (kind gifts from Dr Koichi Suzuki (National Institute of Infectious Diseases, Tokyo, Japan)), HEK293T cells, prostate cancer DU145 cells and PC-3 cells (kind gifts from Dr Akio Matsubara (Hiroshima University)) were maintained in DMEM medium (Nissui Pharmaceutical Co., Tokyo, Japan) supplemented with 10% fetal bovine serum (Biomol, Nuaille, France) and antibiotics. Rat thyroid FRTL-5 cells were kindly provided by the late Dr Leonard Kohn (Ohio University and Edison Biotechnology Institute, OH, USA) and the Interthyr Research Foundation (Baltimore, MD, USA). FRTL-5 cells were cultured in Coon's F-12 medium (Sigma-Aldrich) supplemented with 0.33 mg ml −1 glutamine, MEM non-essential amino acids (ICN Biochemicals, Costa Mesa, CA, USA), 5% newborn bovine serum, 1 mU ml −1 TSH, 10 μg ml −1 insulin, 5 μg ml −1 transferrin and antibiotics. For FRTL-5 cells to become quiescent, the cells were washed twice with Hank’s balanced salt solution (Nissui) and cultures were continued for an additional 24–48 h in starvation medium (Coon's F-12 medium supplemented with 0.33 mg ml −1 glutamine, MEM non-essential amino acids and 0.1% bovine serum albumin). The quiescent FRTL-5 cells were then cultured in starvation medium supplemented with or without 1 mM dibutyryl cAMP for 24 h. In some experiments, the cells were washed three times with Hank’s balanced salt solution and then cultured in starvation medium for 30 min, followed by IGF-I stimulation for indicated durations. HEK293 cells were transfected with plasmids and/or siRNA using Lipofectamine 2000 (Life Technologies, Gaithersburg, MD, USA). The maximum transfection efficiency was about 90%, based on the evaluation using cells transfected with plasmids encoding green fluorescent protein. HEK293T cells were transfected with plasmids using polyethylenimine (Linear, molecular weight 25,000 Da; Polysciences, Warrington, PA, USA) as follows. Subconfluent cells on 60 mm dishes (2 ml of 10% FBS-DMEM) were prepared. Two micrograms of plasmid was mixed with 6 μl of polyethylenimine solution (1 mg ml −1 ) in 200 μl Opti-MEM (Life Technologies). After incubation for 15 min, the mixture was added to cells. Twelve hours later, the culture medium was changed to fresh growth medium and cell culture was continued for 12 h. Cells were then serum starved for 18 h, followed by indicated biochemical experiments. FRTL-5 cells and PC-3 cells were transfected with siRNA using Lipofectamine RNAiMAX (Life Technologies). MS analysis of IRS-2-associated proteins Immunoprecipitates with antibodies against IRS-2 C terminus were subjected to SDS–PAGE, followed by gel staining using SilverQuest (Life Technologies). Gel slices were destained according to the protocols attached to the gel staining kits and then equilibrated with 50 mM NH 4 HCO 3 for 15 min. After the reagent was removed, gel slices were mixed with dehydration buffer (50 mM NH 4 HCO 3 , 50% CH 3 CN) and vortexed for 15 min. After the dehydration procedure was repeated again, gels were dried by vacuum evaporator centrifuge VEC-260 (ASAHI GLASS, Chiba, Japan). Gels were then reswollen in reducing buffer (10 mM dithiothreitol, 25 mM NH 4 HCO 3 ) and incubated for 1 h at 56 °C. After the equal volume of alkylation buffer (55 mM iodoacetamide, 25 mM NH 4 HCO 3 ) was added, the mixtures were shaded and vortexed for 30 min at room temperature. Gels were then equilibrated with 50 mM NH 4 HCO 3 , dehydrated with 50% CH 3 CN and dried by VEC-260 as described above. After reswelling on ice in digestion buffer (10 μg ml −1 Trypsin Gold, Mass Spectrometry Grade (Promega, Madison, WI, USA), 50 mM NH 4 HCO 3 , 5 mM CaCl 2 ), gels were incubated for 16 h at 37 °C. To extract the tryptic peptides, 5% trifluoroacetic acid (TFA) was added and the supernatant was recovered. Gels were then vortexed in 5% TFA/30% CH 3 CN for 5 min and sonicated for 20 min, and the supernatant was recovered. The same procedure was repeated using 5% TFA/50% CH 3 CN and 5% TFA/70% CH 3 CN sequentially. All supernatants were collected and concentrated to 10 μl by VEC-260 and TFA (final concentration, 0.1%) was added to the samples. To desalt the sample, ZipTip μC18 (Millipore) was swollen in 0.1% TFA/50% CH 3 CN and equilibrated with 0.1% TFA/2% CH 3 CN, and the samples were then adsorbed and washed with 0.1% TFA/2% CH 3 CN. The tryptic peptides were eluted with 1 μl of 0.1% TFA/66% CH 3 CN onto a 100-well gold sample plate (Applied Biosystems, Framingham, MA, USA), mixed with 1 μl of matrix solution (10 mg ml −1 α-cyano-4-hydroxy cinnamic acid in 0.2% TFA/60% CH 3 CN) and dried at room temperature. The samples were analysed by matrix-assisted laser desorption/ionization–time-of-flight MS Voyager-DE STR (Applied Biosystems) in peptide-sensitivity reflector mode. The spectra were obtained by the accumulation of 200–1,000 consecutive laser shots and calibrated by mass values of auto-digested trypsin peptides. The mass data were subjected to MASCOT PMF search tools (Matrix Science, London, UK). Pull-down assay Cells were lysed in ice-cold lysis buffer (50 mM Tris-HCl pH 7.4, 150 mM NaCl, 1 mM NaF, 1 mM EDTA, 1 mM EGTA, 1% Triton X-100, 500 μM Na 3 VO 4 , 10 mg ml −1 p -nitrophenyl phosphate, protease inhibitor cocktail (Sigma-Aldrich, P8340)). In pull-down assay, lysates were incubated with 100 pmol of GST-fused proteins for 2 h and then 10 μl of GST–Sepharose beads (GE Healthcare). After 1 h incubation, beads were washed four times with ice-cold lysis buffer and proteins were subjected to SDS–PAGE followed by immunoblotting. Immunoprecipitation and immunoblotting Cells were lysed with ice-cold lysis buffer. The lysates were centrifuged at 15,000 g for 10 min at 4 °C. The protein assay of the supernatant was carried out using a protein assay kit (Bio-Rad, Hercules, CA, USA). Equal amounts of proteins of each sample were mixed with 1/4 volume of 4 × Laemmli’s buffer (0.4 M Tris-HCl pH 6.8, 8% SDS, 20% glycerol, 10% 2-mercaptoethanol, 0.2% bromophenol blue). The mixtures were boiled for 5 min and subjected to SDS–PAGE. In immunoprecipitation, equal amounts of proteins of each sample were mixed with indicated antibodies (their concentrations were as recommended by manufacturers). Samples were incubated at 4 °C for 12 h and then mixed with 10 μl of Protein A-Sepharose or Protein G-Sepharose (GE Healthcare). After the additional incubation for 1 h, precipitates were washed with ice-cold lysis buffer three times and diluted with 1 × Laemmli’s buffer. After boiling for 5 min, the supernatant was subjected to SDS–PAGE. The immunoprecipitation using anti-FLAG antibody-conjugated agarose beads followed by elution with FLAG peptide (Sigma-Aldrich) was performed according to the manufacturer’s recommended protocols. The eluates were mixed with 1/4 volume of 4 × Laemmli’s buffer, boiled for 5 min and subjected to SDS–PAGE. After SDS–PAGE, proteins were transferred onto a polyvinylidene difluoride membrane. The indicated first antibodies and HRP-conjugated second antibodies were hybridized according to standard immunoblotting protocols (their concentrations were as recommended by manufacturers). Chemiluminescence reactions were carried out using SuperSignal West Pico/Femto (Thermo Fisher Scientific, Rockford, IL, USA) and the luminescence was exposed onto X-ray film (X-Omat, Kodak, Tokyo, Japan). Densitometric analysis was carried out using ImageJ 1.43u programme (National Institutes of Health, Bethesda, MD, USA). Uncropped scans of blots are shown in Supplementary Figs 9–13 . In sample preparation for the detection of ubiquitination signals as well as the interaction of IRS-2-Epsin1 (or other ubiquitin-binding proteins), cells were lysed with lysis buffer supplemented with 2 mM N-ethylmaleimide, to inhibit de-ubiquitinating enzymes. In addition, protein samples for the detection of ubiquitination signals were denatured by mixing with 2% SDS and boiling for 5 min, to disassemble protein complex, and then diluted to 20 times by lysis buffer followed by immunoprecipitation. After SDS–PAGE and transfer to a polyvinylidene difluoride membrane, the membrane was denatured by incubating in denaturing buffer (6 M guanidine-HCl, 20 mM Tris-HCl pH7.5, 5 mM β-mercaptoethanol, 1 mM phenylmethyl sulphonyl fluoride) for 30 min and then washed several times with 0.1% Tween20/PBS before immunoblotting using anti-ubiquitin antibody. Cell-free ubiquitination HEK293T cells overexpressing FLAG or FLAG-IRS-2 (one 100-mm culture dish of cells per assay) were lysed and subjected to immunoprecipitation using 20 μl anti-FLAG antibody-conjugated beads (Sigma-Aldrich). Immunoprecipitates on beads were mixed with 150 ng His-human E1 (Biomol, Plymouth, PA, USA), 300 ng His-human UbcH5b (Biomol), 750 ng GST-Nedd4 or GST produced by us, 7.5 μg ubiquitin (Sigma-Aldrich) and 2 mM ATP, in the reaction buffer (25 mM Tris-HCl pH7.5, 120 mM NaCl, 0.5 mM dithiothreitol and 2 mM MgCl 2 ). After the incubation for 2 h at 30 °C, immunoprecipitates were washed with lysis buffer four times, followed by immunoblotting. LC-MS/MS analysis to determine IRS-2 ubiquitination sites FLAG-tagged IRS-2 was immunoprecipitated with anti-FLAG antibody-conjugated beads. The immunoprecipitates were mixed with 100 μl of trypsin solution (10 ng μl −1 Trypsin Gold Mass Spectrometry Grade, 50 mM ammonium bicarbonate, 0.01% RapiGest SF (Waters, Milford, MA, USA)), trypsin and Asp-N solution (10 ng μl −1 Trypsin Gold, 6.6 ng μl −1 Asp-N (Promega), 50 mM ammonium bicarbonate, 0.01% RapiGest SF), or trypsin and chymotrypsin solution (10 ng μl −1 Trypsin Gold, 10 ng μl −1 chymotrypsin (Promega), 100 mM Tris-HCl pH8.0, 10 mM CaCl 2 , 0.01% RapiGest SF). The samples were incubated at 37 °C for 12 h. After a brief centrifugation, supernatants were recovered, mixed with 100 μl of TFA and then desalted using GL-Tip SDB and GL-Tip GC (GL Sciences, Tokyo, Japan). The samples were diluted with IAP buffer (Cell Signaling), mixed with anti-ubiquitin remnant motif antibody-conjugated beads and then incubated at 4 °C for 2 h. The immunoprecipitates were washed with IAP buffer twice and with water three times. Peptides were eluted by 0.15% TFA, desalted with GL-Tip SDB and GL-Tip GC, and then subjected to LC-MS/MS analysis (nano-liquid chromatography column (EASY-nLC 1000, Thermo Fisher Scientific) coupled to Q Exactive mass spectrometer (Thermo Fisher Scientific)) [54] . Data were analysed by Proteome Discoverer software (Thermo Fisher Scientific) and ProteinPilot software (AB SCIEX, Framingham, MA). Peptide quantification was carried out by parallel reaction monitoring, a MS/MS-based quantification method. The extracted peptides were analysed by Q Exactive in targeted MS/MS mode. Raw files were processed by PinPoint software (Thermo Fisher Scientific). Ion chromatograms were extracted with a mass tolerance of 5 p.p.m. The area under the curve of selected fragment ion was calculated. The AUCs of each individual fragment ions were then summed to obtain AUCs at the peptide level [54] . Biotinylation of cell surface proteins Cells were incubated with 1 mg ml −1 NHS-LC biotin (Thermo Fisher Scientific)/PBS for 20 min at 4 °C and then washed twice with 100 mM glycine/PBS. The cells were then lysed with lysis buffer, followed by immunoprecipitation and blotting with HRP-conjugated streptavidin (Sigma-Aldrich) and indicated antibodies. Subcellular fractionation Cells were homogenized in ice-cold detergent-free buffer (40 mM Tris-HCl pH 7.4, 120 mM NaCl, 1 mM EDTA, 1 mM EGTA, 10 mM pyrophosphate, 50 mM NaF, 500 μM Na 3 VO 4 , 10 mg ml −1 p -nitrophenyl phosphate, protease inhibitor cocktail). Samples were then subjected to ultracentrifugation (100,000 g , 1 h). The supernatants were recovered as cytosol fractions. The precipitates were solubilized with lysis buffer as described above (containing 1% Triton X-100), followed by centrifugation (15,000 g , 10 min) and the supernatants were recovered as membrane fractions. Thymidine incorporation into DNA Cells were cultured in 48-well plates or 24-well plates and [ Methyl - 3 H]thymidine (0.3 μCi per well; 1 μCi ml −1 , GE Healthcare) was added to each well for indicated durations. The labelling was stopped by adding 500 μl of 1 M ascorbic acid. The cells were washed twice with ice-cold PBS and twice with ice-cold 10% trichloroacetic acid. Trichloroacetic acid -precipitated materials were solubilized with 250 μl of 0.2 N NaOH/0.1% SDS and mixed into 5 ml clear-sol II (Nakalai tesque). The radioactivity was measured by liquid scintillation counter (Aloka, Tokyo, Japan). Zebrafish experiments Wild-type zebrafish ( Danio rerio ) were kept at 28 °C under a light/dark cycle of 14 and 10 h, and fed twice daily. The wild-type embryos obtained by natural breeding were raised at 28.5 °C and staged [55] . Capped RNAs were synthesized using mMESSAGE mMACHINE Kit (Life Technologies). Venus mRNA (200 pg per embryo), Nedd4-Venus mRNA (1,200 pg per embryo) or 5′-UTR Irs2 -Venus RNA (250 pg per embryo) was co-injected with either control MO or Irs2 MO (4 ng per embryo) into embryos at one- to two-cell stage. Embryos were then placed in embryo-rearing medium [34] and kept at 28.5 °C. Body length and somite number were measured at 22 h post fertilization. Body length was defined as the curvilinear distance from the middle of the otic vesicle to the end of tail through the trunk midline. The expression of Nedd4-Venus was confirmed by fluorescence and immunoblotting. Specific translation block with Irs2 MO were confirmed by the decreases of 5′-UTR Irs2 -Venus fluorescence. All experiments were conducted in accordance with the guidelines approved by the Ethical Committee of Experimental Animal Care at Ocean University of China. Statistical analysis The results shown are the mean±s.d., except for Fig. 7b,c . In Fig. 7b,c , the results are shown as the mean±s.e.m. Data were analysed by Student’s t -test or one-way factorial analysis of variance followed by Tukey–Kramer post-hoc multiple comparison test. P <0.05 was considered statistically significant (shown as ‘*’ in graphs). T.F., H.Y., H.F., H. Kamei (H.K. 1 ), F.H. and S.-I.T. conceived and designed these experiments. T.F., H.Y., H.F., H.K. 1 , F.H., J.L., C.D., Y.S., K.T., S.I. and T.N. performed the experiments. T.F., H.Y., H.F., H.K. 1 , F.H., J.L., C.D., Y.S., K.T., S.I., T.N., K.C., Y.N., H.Kamata (H.K. 2 ), T.A. and S.-I.T. analysed the data and contributed reagents/materials/analysis tools. T.F., H.Y., H.F., H.K. 1 , F.H., C.D. and S.-I.T. wrote the paper. S.-I.T. took the primary responsibility for final content. T.F., H.Y., H.F., H.K. 1 , F.H., C.D., Y.S., K.T., K.C., Y.N., H.K. 2 , T.A. and S.-I.T. read and approved the final manuscript. How to cite this article: Fukushima, T. et al. Nedd4-induced monoubiquitination of IRS-2 enhances IGF signalling and mitogenic activity. Nat. Commun. 6:6780 doi: 10.1038/ncomms7780 (2015).